Errors in the measurement of voltage-activated ion channels in cell-attached patch-clamp recordings Patch-clamp recording techniques have revolutionized understanding of the function and sub-cellular location of ion channels in excitable cells. The cell-attached patch-clamp configuration represents the method of choice to describe the endogenous properties of voltage-activated ion channels in the axonal, somatic and dendritic membrane of neurons, without disturbance of the intracellular milieu. Here, we directly examine the errors associated with cell-attached patch-clamp measurement of ensemble ion channel activity. We find for a number of classes of voltage-activated channels, recorded from the soma and dendrites of neurons in acute brain-slices and isolated cells, that the amplitude and kinetics of ensemble ion channel activity recorded in cell-attached patches is significantly distorted by transmembrane voltage changes generated by the flow of current through the activated ion channels. We outline simple error–correction procedures that allow a more accurate description of the density and properties of voltage-activated channels to be incorporated into computational models of neurons. Voltage-activated ion channels form the electrical excitability of cells. This is of particular relevance in the nervous system in which electrical excitability is a fundamental property of neurons and neuronal circuits. An accurate description of the sub-cellular localization and functional characteristics of voltage-activated channels is therefore essential for an understanding of the operation, and the development of accurate computational models, of central neurons and neural networks [1] , [2] , [3] , [4] . The sub-cellular distribution of voltage-activated channels has been examined using electrophysiological, imaging and immunohistochemical techniques. The use of channel-type-specific antibodies coupled with fluorescent reporters, however, do not describe quantitatively the density of ion channels, which is only achievable using specialized, high sensitivity, quantitative electron microscopic immunogold staining methods [5] . In contrast, electrophysiological techniques provide valuable tools to investigate the functional properties and quantify the sub-cellular density of ion channels [6] . However, many electrophysiological approaches, such as whole-cell patch-clamp recordings do not accurately describe the macroscopic properties of voltage-activated channels [7] , [8] , [9] . The functional properties and sub-cellular densities of voltage-activated channels in the axonal, somatic and dendritic membrane of neurons have been more successfully investigated using cell-attached and cell-free patch-clamp approaches [6] , [10] , [11] , [12] , [13] , [14] , [15] , [16] , [17] , [18] , [19] , [20] , [21] , [22] , [23] , [24] , [25] , [26] , [27] . The cell-attached configuration is unique among these recording approaches, as it does not perturb the intracellular milieu or rely on the excision of the membrane, which potentially disrupts the function of ion channels [6] , [28] , [29] , [30] . Moreover, voltage-activated channels in the tip of the patch-clamp electrode are subject to near-perfect extracellular voltage control, because of the tight electrical seal between the recording electrode and the membrane [6] . Pioneering work, however, demonstrated that single voltage-activated ion channel events could be distorted when recorded in cell-attached patches from isolated cells or membrane vesicles [31] , [32] , [33] . Such distortion was predicted, although not directly observed, to arise because of the generation of intracellular voltage changes evoked by current flow through activated voltage-activated ion channels [31] , [32] , [33] ; with the magnitude of voltage changes, and so the distortion of the waveform of ion channel activity formed as a consequence of the very high apparent input resistance (>5 GΩ) of isolated cells and membrane vesicles, as dictated by Ohm's law. Subsequent studies using cell-attached recording techniques to study the density and properties of ensemble voltage-activated channel activity in central neurons, which typically exhibit lower apparent input resistance than isolated cells and membrane vesicles, have largely neglected this and other [12] potential sources of error. In this study, we report errors in the measurement of the sub-cellular density and functional properties of voltage-activated ion channels in cell-attached recordings from the soma and dendrites of central neurons maintained in acute brain-slices. We directly demonstrate that such errors arise because of transmembrane voltage changes generated by the activation of voltage-activated channels in the tip of the patch-clamp pipette and outline simple procedures that allow the correction of measurement errors. Potassium channel activity drives neuronal output During the study of the sub-cellular distribution of voltage-activated ion channels in central neurons, we sought to determine the resting membrane potential (RMP) of thalamocortical (TC) neurons of the dorsal lateral nucleus using non-invasive procedures. One commonly used technique is to measure the reversal potential of ensemble potassium channel activity recorded in cell-attached patches [34] , [35] . To do this we made tight-seal (7.1±1.2 GΩ; n =28), cell-attached voltage-clamp (v-c) recordings with pipettes containing a potassium-based filling solution from the somata of visually identified TC neurons maintained in acute brain-slices at room temperature ( Fig. 1 ). In response to rapid voltage ramps (2 Vs −1 , V H =0 mV, ramp from 100 to −200 mV) large potassium currents were generated with a characteristic voltage dependence ( Fig. 1a,b ; n =28) (ref. 34 ). To our surprise we observed that in the majority of recordings ( n =20) a period of action potential firing was generated following the termination of extracellular voltage ramps ( Fig. 1a,b ). Action potentials were typically generated as high frequency bursts and invariably followed the offset of the voltage ramp applied to the cell-attached pipette ( Fig. 1b , inset, Fig. 1c ; on average 2.7±0.3 action potentials per burst; n =654). The time-locked nature of action potential burst firing suggested their generation in response to the cell-attached voltage ramps or the evoked ensemble potassium channel activity. Previous investigations have, however, suggested that ensemble potassium channel activity does not lead to a change in the intracellular membrane potential, thus allowing the non-invasive measurement of the neurons RMP [34] , [36] . To directly explore how action potential firing was generated, we made simultaneous whole-cell and cell-attached recordings from the somata of TC neurons with electrodes filled with identical potassium-based solutions, and evoked ensemble potassium channel activity in response to extracellularly applied voltage ramps ( Fig. 1d ). Notably, we observed a dramatic hyperpolarization of the whole-cell recorded membrane potential that evolved with a time course similar to that of the potassium current simultaneously recorded in the cell-attached patch ( Fig. 1d ). The evoked voltage responses were followed by a period of repolarization and the generation of low threshold calcium potentials [37] crowned by the burst firing of action potentials ( Fig. 1d ; n =22). The peak amplitude of the recorded membrane potential change was related to the magnitude of ensemble potassium channel activity recorded simultaneously in the cell-attached configuration ( Fig. 1e ). Furthermore, we found that when cell-attached recordings were made with pipettes filled with a sodium-based solution that contained blockers of potassium channels, the cell-attached voltage ramp evoked little channel activity or intracellular voltage change ( Fig. 1e ; grey symbols). These data suggest that the evoked ensemble potassium channel activity, and not the applied extracellular voltage ramp, acts to hyperpolarize the membrane potential. To examine this idea, we injected negative going current ramps through the recording electrode during whole-cell current-clamp (c-c) recordings with amplitude and time course similar to that of ensemble potassium channel activity ( Fig. 1f ; ramp amplitude −227±19 pA; ramp slope=2 nA s −1 ; ramp duration=100 ms). Negative current ramps generated hyperpolarizing voltage responses similar to those generated by cell-attached currents, which consistently evoked low threshold calcium potentials crowned by the burst firing of action potentials ( Fig. 1f ; peak voltage change=−33.5±1.1 mV; n =9). Taken together, these data suggest that ensemble potassium channel activity generated in cell-attached patches leads to dramatic membrane hyperpolarization of TC neurons, bringing into question the use of this technique to non-invasively record the RMP of central neurons. Indeed, the RMP of TC neurons recorded in the whole-cell configuration was significantly different to that predicted by the reversal potential of ensemble potassium channel activity [34] ( Fig. 1g ; Supplementary Fig. S1 ; recorded: 56.8±0.8 mV; predicted: 58.3±0.7 mV; P <0.0001; n =28). 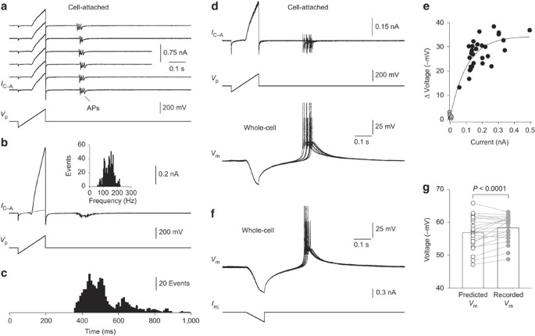Figure 1: Ensemble potassium channel activity in cell-attached patches triggers action potential firing. (a) Tiled consecutive traces of action potential (AP) firing triggered by ensemble potassium channel activity in a cell-attached (IC-A) patch made from the soma of a visually identified thalamocortical (TC) neuron. The lower trace shows the voltage command ramp (Vp). (b) Digital average (n=30 responses) of ensemble potassium channel activity evoked in the cell-attached patch shown ina. The fitted grey line represents the leak current. The inset shows the instantaneous AP firing frequency. (c) Post-stimulus time histogram of AP firing generated by ensemble potassium channel activity in cell-attached patches (data pooled from 20 neurons). (d) Simultaneous cell-attached (IC-A) and whole-cell current-clamp (Vm) recording from the soma of a TC neuron. Five consecutive traces have been overlain. (e) Relationship between the peak amplitude of ensemble potassium channel activity and intracellular voltage responses, for cell-attached pipettes filled with a potassium-based solution (black symbols) or a solution that included the potassium channel blockers 4-aminopyridine and tetraethylammonium (grey symbols). Data have been fit by an exponential function (line). (f) Voltage responses (Vm) evoked by the injection of a ramp of negative current through the recording electrode (Iinj) during somatic whole-cell current-clamp recording. Five consecutive traces have been overlain. (g) Resting membrane potential of TC neurons determined by whole-cell current-clamp recording (recorded) or predicted by measurement of the reversal potential of ensemble potassium channel activity in cell-attached patches (n=28). Data were compared with a paired Student'st-test. Figure 1: Ensemble potassium channel activity in cell-attached patches triggers action potential firing. ( a ) Tiled consecutive traces of action potential (AP) firing triggered by ensemble potassium channel activity in a cell-attached ( I C-A ) patch made from the soma of a visually identified thalamocortical (TC) neuron. The lower trace shows the voltage command ramp ( V p ). ( b ) Digital average ( n =30 responses) of ensemble potassium channel activity evoked in the cell-attached patch shown in a . The fitted grey line represents the leak current. The inset shows the instantaneous AP firing frequency. ( c ) Post-stimulus time histogram of AP firing generated by ensemble potassium channel activity in cell-attached patches (data pooled from 20 neurons). ( d ) Simultaneous cell-attached ( I C-A ) and whole-cell current-clamp ( V m ) recording from the soma of a TC neuron. Five consecutive traces have been overlain. ( e ) Relationship between the peak amplitude of ensemble potassium channel activity and intracellular voltage responses, for cell-attached pipettes filled with a potassium-based solution (black symbols) or a solution that included the potassium channel blockers 4-aminopyridine and tetraethylammonium (grey symbols). Data have been fit by an exponential function (line). ( f ) Voltage responses ( V m ) evoked by the injection of a ramp of negative current through the recording electrode ( I inj ) during somatic whole-cell current-clamp recording. Five consecutive traces have been overlain. ( g ) Resting membrane potential of TC neurons determined by whole-cell current-clamp recording (recorded) or predicted by measurement of the reversal potential of ensemble potassium channel activity in cell-attached patches ( n =28). Data were compared with a paired Student's t -test. Full size image Impact of voltage changes on ion channel activity Next, we explored the functional consequences of transmembrane voltage changes evoked by ensemble voltage-activated channel activity in cell-attached patches. We reasoned that transmembrane voltage changes could affect the amplitude and/or shape of the ensemble channel activity recorded in cell-attached patches, unless the intracellular voltage was held constant. To test this we evoked voltage-activated channel activity in cell-attached patches and made simultaneous somatic whole-cell v-c or c-c recordings from inhibitory interneurons of the stratum radiatum (SR) of the CA1 region of the hippocampus, the cell-type used to establish the utility of cell-attached patch-clamp techniques to non-invasively measure the RMP [34] and TC neurons maintained at room temperature ( Fig. 2 ; SR interneurons third quadrant input resistance: maximum=448.8±38.2 MΩ, minimum=215.2±36.6 MΩ; TC neurons third quadrant input resistance: maximum=357.8±20.1 MΩ, minimum=72.1±10.5 MΩ). When the intracellular potential was voltage-clamped at the RMP the activation of cell-attached ensemble potassium channel activity resulted in the generation of an outward current in the whole-cell configuration ( Fig. 2a,b ). The peak amplitude and time course of the whole-cell recorded current closely resembled that of the cell-attached current, but was of opposite polarity; however, by convention, cell-attached currents have been inverted for illustration ( Fig. 2a ). These data indicate that the activation of ensemble channel activity in cell-attached patches represents a transmembrane current that can be recorded at the whole-cell level. To explore how evoked transmembrane voltage changes impacted on the characteristics of cell-attached currents, we switched the whole-cell recording amplifier to c-c mode, thus allowing the intracellular membrane potential to freely vary, as occurs in the unperturbed state. Under these conditions, the peak amplitude and time-integral of cell-attached currents were distorted in both SR interneurons and TC neurons ( Fig. 2a,c ; peak amplitude SR interneurons: v-c=174.3±33.7 pA; c-c=135.8±27.0 pA; P <0.001; n =11; TC neurons: v-c=226.0±24.5 pA; c-c=180.7±18.2 pA; P <0.002; n =18). This arose because of the prominent transmembrane voltage changes evoked by ensemble potassium channel activity in these neuronal classes ( Figs 1e and 2d ). 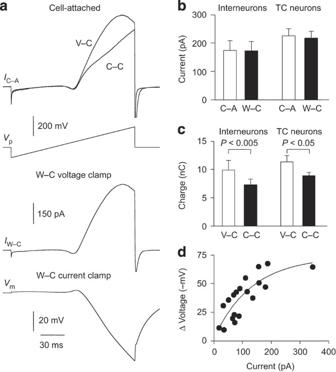Figure 2: Ensemble potassium channel activity in cell-attached patches generates whole-cell currents. (a) Simultaneous whole-cell recording of ensemble potassium channel activity generated in a cell-attached patch (IC-A) under whole-cell voltage-clamp (v-c) or current-clamp (c-c) conditions from the soma of a stratum radiatum interneuron of the CA1 region of the hippocampus. Note that under whole-cell v-c, an outward current with kinetics and amplitude similar to the cell-attached current was recorded (IW-C). When the whole-cell voltage was not clamped, under c-c recording conditions, the amplitude and shape of the cell-attached current was modified and a prominent hyperpolarizing voltage response recorded intracellularly (Vm). The pipette voltage command ramp is shown (VP). (b) The peak amplitude of outward currents gated by ensemble potassium channel activity is similar when recorded at the cell-attached (C-A) and whole-cell (W-C) level in stratum radiatum interneurons (n=11) and thalamocortical (TC) neurons (n=18). (c) The charge of ensemble potassium channel activity in cell-attached patches is significantly different when the simultaneous whole-cell recording is configured in v-c or c-c mode. (d) Relationship between the amplitude of potassium currents in cell-attached patches and hyperpolarizing voltage changes in stratum radiatum interneurons. Data have been fit by a single exponential function (line). Pooled data are shown as mean±s.e.m., statistical significance was determined with a paired Student'st-test. Figure 2: Ensemble potassium channel activity in cell-attached patches generates whole-cell currents. ( a ) Simultaneous whole-cell recording of ensemble potassium channel activity generated in a cell-attached patch ( I C-A ) under whole-cell voltage-clamp (v-c) or current-clamp (c-c) conditions from the soma of a stratum radiatum interneuron of the CA1 region of the hippocampus. Note that under whole-cell v-c, an outward current with kinetics and amplitude similar to the cell-attached current was recorded ( I W-C ). When the whole-cell voltage was not clamped, under c-c recording conditions, the amplitude and shape of the cell-attached current was modified and a prominent hyperpolarizing voltage response recorded intracellularly ( V m ). The pipette voltage command ramp is shown ( V P ). ( b ) The peak amplitude of outward currents gated by ensemble potassium channel activity is similar when recorded at the cell-attached (C-A) and whole-cell (W-C) level in stratum radiatum interneurons ( n =11) and thalamocortical (TC) neurons ( n =18). ( c ) The charge of ensemble potassium channel activity in cell-attached patches is significantly different when the simultaneous whole-cell recording is configured in v-c or c-c mode. ( d ) Relationship between the amplitude of potassium currents in cell-attached patches and hyperpolarizing voltage changes in stratum radiatum interneurons. Data have been fit by a single exponential function (line). Pooled data are shown as mean±s.e.m., statistical significance was determined with a paired Student's t -test. Full size image Errors in the measurement of ion channel density To examine whether the generation of transmembrane voltage changes distorts the measurement of the density of ion channels in cell-attached patches, we examined pharmacologically isolated, leak-subtracted, cell-attached potassium currents evoked by simple voltage steps in TC neurons ( Fig. 3 ) and dopaminergic neurons of the substantia nigra, which display prominent voltage-activated potassium channel activity [25] ( Supplementary Fig. S2 ). First, we made simultaneous somatic cell-attached ( V H =0 mV) and whole-cell v-c recordings from TC neurons maintained at room temperature. When the intracellular voltage was held constant, at the RMP, potassium channels in cell-attached patches typically gated a fast rising, but slowly decaying current ( Fig. 3a ). However, in the same patches, when the intracellular voltage was not clamped, in c-c mode, potassium currents were characterized by a prominent early transient component, which rapidly decayed to steady state, leading to a dramatic acceleration of the decay time-constant when compared with whole-cell v-c recording conditions ( Fig. 3a ; v-c=218.6±38.4 ms; c-c=57.2±6.1 ms; n =31; P <0.001). To quantify this difference, we plotted the relationship between the amplitude of the cell-attached current and the whole-cell recorded v-c current, finding the expected linear relationship when the current was measured at peak amplitude or steady state ( Fig. 3b,c ). However, when the intracellular voltage was allowed to vary freely in c-c mode, we found a reduction of the peak amplitude of the cell-attached current ( Fig. 3b ; v-c=208.4±19.8 pA; c-c=185.2±17.4 pA; n =32; P <0.001). This difference was increased when the cell-attached potassium current was measured at steady state, revealing a large error in channel density measurement ( Fig. 3c , v-c=161.0±15.1 pA; c-c=107.0±7.8 pA; n =32; P <0.001). The distortion of cell-attached currents at peak and steady state was reflected by a difference in the magnitude of whole-cell recorded voltage deviations measured at these time points ( Fig. 3d ). These data suggest that whole-cell voltage responses evolve during the course of the cell-attached potassium current, presumably due to the charging of the neuronal membrane. 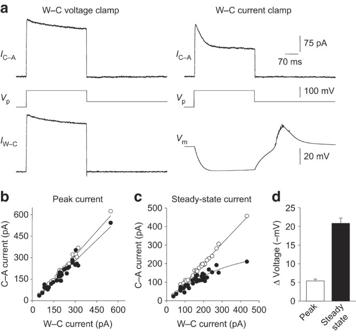Figure 3: The surface density of voltage-activated potassium channels is under-estimated in cell-attached recordings. (a) Leak-subtracted ensemble potassium channel activity (IC-A) generated in response to a voltage step protocol (Vp) during simultaneous whole-cell voltage- (left) and current-clamp recording from the soma of a thalamocortical neuron. Cell-attached currents were accompanied by the generation of a whole-cell recorded outward current (IW-C) or a hyperpolarizing voltage response (Vm) under voltage- or current-clamp conditions, respectively. (b,c) Linear relationship between the amplitude of ensemble potassium channel activity recorded in cell-attached patches and as whole-cell current (open symbols) when measured at peak (b) and steady state (c). Filled symbols illustrate the magnitude of ensemble potassium channel activity recorded from the same patches under whole-cell current-clamp conditions, and are plotted with reference to the value of whole-cell current recorded under voltage-clamp mode for each patch. Data have been fit by linear regression or with an exponential function (lines). (d) The amplitude of intracellular voltage responses recorded under whole-cell current-clamp generated by ensemble potassium channel activity in cell-attached patches. Voltage responses were measured at time points corresponding to the peak amplitude (peak) of the cell-attached current or at steady state. Pooled data (n=32) are represented as mean±s.e.m. Figure 3: The surface density of voltage-activated potassium channels is under-estimated in cell-attached recordings. ( a ) Leak-subtracted ensemble potassium channel activity ( I C-A ) generated in response to a voltage step protocol ( V p ) during simultaneous whole-cell voltage- (left) and current-clamp recording from the soma of a thalamocortical neuron. Cell-attached currents were accompanied by the generation of a whole-cell recorded outward current ( I W-C ) or a hyperpolarizing voltage response ( V m ) under voltage- or current-clamp conditions, respectively. ( b , c ) Linear relationship between the amplitude of ensemble potassium channel activity recorded in cell-attached patches and as whole-cell current (open symbols) when measured at peak ( b ) and steady state ( c ). Filled symbols illustrate the magnitude of ensemble potassium channel activity recorded from the same patches under whole-cell current-clamp conditions, and are plotted with reference to the value of whole-cell current recorded under voltage-clamp mode for each patch. Data have been fit by linear regression or with an exponential function (lines). ( d ) The amplitude of intracellular voltage responses recorded under whole-cell current-clamp generated by ensemble potassium channel activity in cell-attached patches. Voltage responses were measured at time points corresponding to the peak amplitude (peak) of the cell-attached current or at steady state. Pooled data ( n =32) are represented as mean±s.e.m. Full size image To directly test this idea, we examined whether the amplitude and shape of voltage responses generated by ensemble channel activity could explain the distortion of the amplitude and time course of potassium currents recorded in cell-attached patches. To do this we multiplied the waveform of ensemble potassium channel activity recorded in each cell-attached patch under simultaneous whole-cell v-c conditions with a voltage command waveform composed of the addition of the voltage command step and the intracellular voltage deviation recorded under whole-cell c-c conditions. We predicted that this voltage waveform approximates the transmembrane voltage change apparent between the tip of the cell-attached patch-clamp electrode and the cell interior that occurs in the unperturbed state. The product of transmembrane voltage change and the cell-attached current, expressed in units of power, recorded under whole-cell v-c should therefore resemble the amplitude and time course of the cell-attached current recorded under whole-cell c-c conditions. We found that such transmembrane voltage corrected cell-attached waveforms were nearly identical to the waveforms recorded under whole-cell c-c conditions ( Fig. 4a,b ). When data were pooled across experiments, we found no difference between the area and kinetics of corrected and c-c recorded waveforms ( Fig. 4c,d ). These data directly show that the intracellular voltage deviations generated by ensemble channel activity explain differences in the amplitude and kinetics of ensemble potassium channel activity recorded in cell-attached patches under whole-cell v-c and c-c recording conditions. Moreover they suggest that errors apparent in cell-attached recordings are formed by intracellular voltage responses, which are dependent on the amplitude and kinetics of the ensemble potassium current generated in the cell-attached patch and the apparent input resistance of the recorded neuron. As the apparent input resistance of central neurons is temperature dependent, decreasing with increasing temperature [38] , [39] , [40] , we explored whether errors in the measurement of ensemble potassium channel activity were extant when recordings were made from TC neurons at near physiological temperatures (35–37 °C). Under these conditions, cell-attached potassium currents evoked large intracellular voltage deviations when the whole-cell recording electrode was configured in c-c mode (peak: −17.8±1.8 mV; steady state: −13.8±1.3 mV), despite the lower apparent input resistance of TC neurons ( Supplementary Fig. S3 ; third quadrant input resistance: maximum=226.8±21.3 MΩ, minimum=56.1±6.7 MΩ; n =15). When the intracellular membrane potential was voltage-clamped the magnitude and time course of ensemble potassium channel activity in cell-attached patches was transformed, resulting in a significant increase in their charge (c-c: 17.3±2.1 pC; v-c: 23.5±3.0 pC; P <0.001; n =15). These data indicate that intracellular voltage perturbations result in a measurement error of the charge of ensemble potassium channel activity in cell-attached patches of 24.4±4.1% at near physiological temperature and 28.1±1.9% at room temperature ( Supplementary Fig. S3 ). 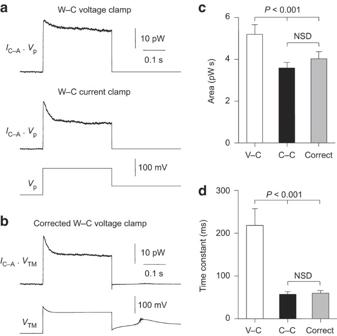Figure 4: Transmembrane voltage responses control the time course of ensemble potassium channel activity in cell-attached patches. (a) The time course of waveforms calculated by multiplying cell-attached leak-subtracted potassium currents by the pipette command voltage (VP) during simultaneous whole-cell (W-C) voltage-clamp (v-c) and current-clamp (c-c) recording from the soma of a thalamocortical neuron. (b) For the same patch, a transmembrane potential corrected waveform was calculated by multiplying the cell-attached current recorded under whole-cell v-c by the estimated transmembrane voltage change that occurred under whole-cell c-c (VTM). Transmembrane voltage was calculated by the addition of the pipette command voltage and the intracellular voltage deviation recorded under whole-cell c-c. Note the similarity of this waveform to that directly recorded under whole-cell c-c conditions (a). (c,d) The area (c) and decay time constant (d) of transmembrane corrected (correct) waveforms are not significantly different (NSD) from those directly recorded under whole-cell c-c conditions. The area and decay time constant of waveforms recorded under whole-cell voltage- and current-clamp conditions are, however, significantly different. Pooled data (n=32) are presented as mean±s.e.m. and statistical significance determined with analysis of variance. Figure 4: Transmembrane voltage responses control the time course of ensemble potassium channel activity in cell-attached patches. ( a ) The time course of waveforms calculated by multiplying cell-attached leak-subtracted potassium currents by the pipette command voltage ( V P ) during simultaneous whole-cell (W-C) voltage-clamp (v-c) and current-clamp (c-c) recording from the soma of a thalamocortical neuron. ( b ) For the same patch, a transmembrane potential corrected waveform was calculated by multiplying the cell-attached current recorded under whole-cell v-c by the estimated transmembrane voltage change that occurred under whole-cell c-c ( V TM ). Transmembrane voltage was calculated by the addition of the pipette command voltage and the intracellular voltage deviation recorded under whole-cell c-c. Note the similarity of this waveform to that directly recorded under whole-cell c-c conditions ( a ). ( c , d ) The area ( c ) and decay time constant ( d ) of transmembrane corrected (correct) waveforms are not significantly different (NSD) from those directly recorded under whole-cell c-c conditions. The area and decay time constant of waveforms recorded under whole-cell voltage- and current-clamp conditions are, however, significantly different. Pooled data ( n =32) are presented as mean±s.e.m. and statistical significance determined with analysis of variance. Full size image Next, we explored whether transmembrane voltage changes distort the measurement of inward currents recorded in cell-attached patches. The cell-attached patch-clamp configuration has recently been used to measure the sub-cellular density and properties of HCN channels in central neurons [13] , [15] , [20] , [22] , [26] , [41] , [42] , as this technique does not disturb the intracellular levels of cyclic nucleotides, which modulate the activation of HCN channels [43] , [44] . To examine cell-attached measurement errors of a single molecularly identified channel-type, we expressed HCN1 channels in HEK293T cells. We made simultaneous whole-cell and cell-attached recording from the cell body of HEK293T cells maintained at room temperature ( Fig. 5 ; maximum first quadrant input resistance=672±124 MΩ). When the intracellular membrane potential of HEK293T cells was voltage-clamped at a potential close to the RMP ( V H whole-cell=−40 mV), the delivery of a 100 mV voltage command step to the cell-attached pipette evoked a slow inward current, which was mirrored as a whole-cell current ( Fig. 5a ; V H cell-attached=−40 mV). In contrast when the whole-cell recording was placed in c-c mode, and the membrane potential set to −40 mV, the amplitude of the cell-attached current was dramatically reduced, and the activation kinetics accelerated ( Fig. 5a–e ). Under these conditions ensemble HCN1 channel activity in cell-attached patches generated a depolarizing intracellular voltage change ( Fig. 5b ; 14.5±1.6 mV; n =19). 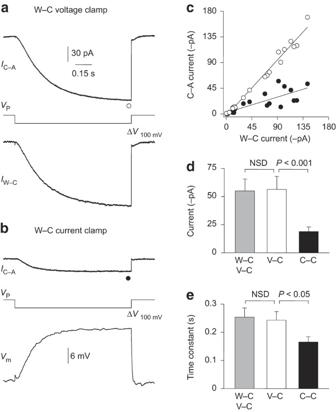Figure 5: HCN1 channel surface density is under-estimated in cell-attached patches. (a) Simultaneous recording of ensemble HCN1 channel activity in a cell-attached patch (IC-A) under whole-cell voltage-clamp (IW-C) from the cell body of a HEK293T cell. The cell-attached pipette command voltage is shown (VP). (b) Simultaneous recording from the same patch under whole-cell current-clamp conditions. (c) Linear relationship between the amplitude of ensemble HCN1 channel activity recorded in cell-attached patches (n=21) and as whole-cell current, under whole-cell voltage-clamp recording conditions (open symbols). Filled symbols illustrate the magnitude of ensemble HCN1 channel activity recorded from the same patches under whole-cell current-clamp conditions, and are plotted with reference to the value of whole-cell current recorded under voltage-clamp mode for each patch. Data have been fit by linear regression or with an exponential function (lines). (d,e) Pooled data show that the steady-state amplitude (d) and activation time constant (e) of ensemble HCN1 channel activity in cell-attached patches (v-c) are not significantly different (NSD) to those simultaneously recorded under whole-cell voltage-clamp (W-C v-c,n=21). In contrast, the amplitude of HCN1 channel activity recorded under whole-cell current-clamp (c-c,n=19) conditions is significantly depressed (d) and the activation time constant accelerated (e). Pooled data are presented as mean±s.e.m. and statistical significance determined with analysis of variance. Figure 5: HCN1 channel surface density is under-estimated in cell-attached patches. ( a ) Simultaneous recording of ensemble HCN1 channel activity in a cell-attached patch ( I C-A ) under whole-cell voltage-clamp ( I W-C ) from the cell body of a HEK293T cell. The cell-attached pipette command voltage is shown ( V P ). ( b ) Simultaneous recording from the same patch under whole-cell current-clamp conditions. ( c ) Linear relationship between the amplitude of ensemble HCN1 channel activity recorded in cell-attached patches ( n =21) and as whole-cell current, under whole-cell voltage-clamp recording conditions (open symbols). Filled symbols illustrate the magnitude of ensemble HCN1 channel activity recorded from the same patches under whole-cell current-clamp conditions, and are plotted with reference to the value of whole-cell current recorded under voltage-clamp mode for each patch. Data have been fit by linear regression or with an exponential function (lines). ( d , e ) Pooled data show that the steady-state amplitude ( d ) and activation time constant ( e ) of ensemble HCN1 channel activity in cell-attached patches (v-c) are not significantly different (NSD) to those simultaneously recorded under whole-cell voltage-clamp (W-C v-c, n =21). In contrast, the amplitude of HCN1 channel activity recorded under whole-cell current-clamp (c-c, n =19) conditions is significantly depressed ( d ) and the activation time constant accelerated ( e ). Pooled data are presented as mean±s.e.m. and statistical significance determined with analysis of variance. Full size image To further understand measurement errors of the density of HCN1 channels, we constructed steady-state activation curves ( Fig. 6 ; n =9). We found, under simultaneous whole-cell v-c recording conditions that the activation kinetics of ensemble HCN1 channel activity quickened and the amplitude increased as the magnitude of the cell-attached voltage command step was increased, consistent with previous reports [45] ( Fig. 6a ). In contrast, under whole-cell c-c recording conditions the activation of ensemble HCN1 channel was significantly perturbed across the voltage range tested, exhibiting accelerated activation kinetics and reduced steady-state amplitude ( Fig. 6b , Supplementary Fig. S4 ). These effects were accompanied by the generation of a depolarizing intracellular voltage response, which was linearly related to the amplitude of ensemble HCN1 channel activity, when measured at steady state ( Fig. 6b,c ; n =9). This data suggest that the generation of depolarizing voltage responses act to decrease the transmembrane voltage sensed by HCN1 channels, and so removes the signal, transmembrane hyperpolarization, required to gate this channel type. To test this, we plotted the steady-state amplitude of ensemble HCN1 channel activity in cell-attached patches recorded under c-c conditions as a function of the predicted transmembrane voltage change (voltage command step plus the intracellular voltage deviation recorded under whole-cell c-c conditions). The calculated voltage–current relationship exhibited a shape similar to that of ensemble HCN1 channel activity directly observed under whole-cell v-c recording conditions ( Fig. 6d , compare open and grey symbols). 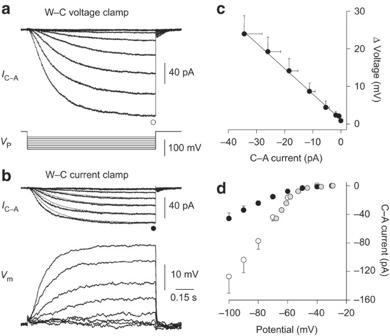Figure 6: The activation properties of HCN1 channels are altered by transmembrane voltage changes. (a) Voltage-dependent activation of ensemble HCN1 channel activity in cell-attached patches (IC-A) recorded under simultaneous whole-cell (W-C) voltage-clamp from a HEK293T cell. The cell-attached voltage command is shown (Vp). (b) Under whole-cell current-clamp conditions the amplitude of the cell-attached current is decreased (black, top traces). Under these conditions the activation kinetics are accelerated, an effect shown by the overlay of a scaled version of traces recorded under whole-cell voltage-clamp (grey traces). The lower traces show the membrane potential depolarization (Vm) evoked by ensemble channel activity. (c) Intracellular voltage change generated by ensemble HCN1 channel activity. Pooled data (n=9) are presented as mean±s.e.m. and have been fit by linear regression (line). (d) Steady-state voltage–current relationship of ensemble HCN1 channel activity in cell-attached patches under whole-cell voltage- (black symbols) and current-clamp (open symbols) conditions. Grey symbols show the predicted voltage-current relationship when cell-attached currents recorded under whole-cell current-clamp are plotted as a function of the calculated transmembrane potential. Pooled data (n=9) are presented as mean±s.e.m. Figure 6: The activation properties of HCN1 channels are altered by transmembrane voltage changes. ( a ) Voltage-dependent activation of ensemble HCN1 channel activity in cell-attached patches ( I C-A ) recorded under simultaneous whole-cell (W-C) voltage-clamp from a HEK293T cell. The cell-attached voltage command is shown ( V p ). ( b ) Under whole-cell current-clamp conditions the amplitude of the cell-attached current is decreased (black, top traces). Under these conditions the activation kinetics are accelerated, an effect shown by the overlay of a scaled version of traces recorded under whole-cell voltage-clamp (grey traces). The lower traces show the membrane potential depolarization ( V m ) evoked by ensemble channel activity. ( c ) Intracellular voltage change generated by ensemble HCN1 channel activity. Pooled data ( n =9) are presented as mean±s.e.m. and have been fit by linear regression (line). ( d ) Steady-state voltage–current relationship of ensemble HCN1 channel activity in cell-attached patches under whole-cell voltage- (black symbols) and current-clamp (open symbols) conditions. Grey symbols show the predicted voltage-current relationship when cell-attached currents recorded under whole-cell current-clamp are plotted as a function of the calculated transmembrane potential. Pooled data ( n =9) are presented as mean±s.e.m. Full size image Next, we explored whether the measurement of native HCN channels was similarly affected. Cell-attached recording techniques have been used to demonstrate that HCN channels are expressed at high densities in the apical dendritic tree of cortcial pyramidal neurons [13] , [15] , [22] , [26] , [42] . To explore the magnitude of intracellular voltage deviations generated by the activation of dendritic HCN channels, we made simultaneous cell-attached v-c ( V H =−20 mV) and whole-cell c-c recordings from apical dendritic sites of neocortical layer 5 pyramidal neurons, with closely spaced electrodes, at room temperature ( Fig. 7 ; distance between electrodes 4 to 12 μm; distance from the soma 200 to 850 μm; n =18). We found a roughly linear relationship between the magnitude of ensemble HCN channel activity recorded in cell-attached patches and intracellular depolarizing voltage deviations, with a slope of 4.7 mV per 100 pA ( Fig. 7a,b ). Notably, when recordings were made at near physiological temperatures, the slope of this relationship was reduced to 2.3 mV per 100 pA ( Fig. 7b ; n =22). As the apparent input resistance at apical dendritic trunk sites is site-independent in layer 5 pyramidal neurons [46] , the slope of this relationship is formed by the site-dependent increase in the density of HCN channels at remote apical dendritic sites [47] . The reduction of the slope of this relationship could largely be accounted for by the decrease in the apparent input resistance at dendritic sites at near physiological temperature (maximum first quadrant apparent input resistance: room: 48.9±7.5 MΩ, n =13; physiological: 24.1±2.6 MΩ; n =8). The magnitude of intracellular voltage deviations evoked at apical dendritic sites increased linearly with the magnitude of ensemble HCN channel activity during the construction of activation curves ( Fig. 7c,d ). Notably, in some recordings, voltage deviations generated at apical dendritic sites were of sufficient magnitude to depolarize the neuron to action potential initiation threshold ( Fig. 7c ). In contrast, the amplitude of intracellular voltage deviations measured at a time point corresponding to the peak amplitude of ensemble HCN channel tail currents were of small amplitude ( Fig. 7c,d ). HCN channel tail currents represent the flow of current at a given voltage during channel deactivation, and are typically used for the construction of activation curves. Because of the intracellular voltage deviations evoked by ensemble HCN channel activity in dendritic cell-attached patches, we re-examined the voltage dependence of HCN channel activation. Using the recorded dendritic whole-cell membrane potential, and the cell-attached pipette potential we were able to calculate the activation curve of ensemble HCN channel activation for each patch either using the cell-attached pipette potential with reference to the RMP (as is done by standard) or following correction for the change in transmembrane voltage produced by ensemble channel activity. We found for each cell-attached patch examined that the voltage at half-maximal activation ( V 1/2 ) and the steepness of the activation curve, when fit with a single Boltzmann function, were significantly changed by this correction procedure (average values from pooled data: uncorrected: V 1/2 =−90.8±2.1 mV, steepness=12.0±0.7; corrected: V 1/2 =−87.9±1.6 mV, steepness=10.8±0.5; n =7; P <0.05). Thus, we were able to calculate, from pooled data, the undistorted activation curve of dendritic HCN channels ( Fig. 7e ). 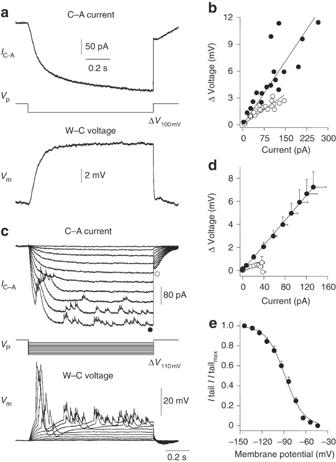Figure 7: Measurement errors of dendritic HCN channels in cell-attached patches. (a) Intracellular voltage change (Vm) evoked by ensemble HCN channel activity (IC-A) simultaneously recorded from the apical dendrite of a layer 5 pyramidal neuron (840 μm from the soma, separation between cell-attached and whole-cell pipette=10 μm). (b) Linear relationship between the amplitude of ensemble HCN channel activity in cell-attached patches and intracellular depolarization at apical dendritic sites of layer 5 pyramidal neurons. Data were gathered at room (23–24 °C, filled symbols) or near physiological (35–37 °C, open symbols) temperatures, and were fit by linear regression (lines). (c) Voltage-dependent activation of ensemble HCN channel activity (IC-A) in a cell-attached patch recorded from the apical dendrite of a layer 5 pyramidal neuron (850 μm from the soma). The lower traces show the intracellular voltage responses simultaneously recorded under whole-cell current-clamp (Vm; 9 μm separation between pipettes). Note the generation of AP firing. (d) Pooled data demonstrating the linear relationship between HCN channel activity in cell-attached patches and intracellular depolarization, when measured at steady-state (filled symbols, fit by linear regression, line), but the minimal voltage deviation apparent at the peak of HCN tail currents (open symbols). Pooled data (n=7) represent mean±s.e.m. (e) Transmembrane voltage corrected activation curve of apical dendritic HCN channels. Pooled data (n=7, mean±s.e.m.) have been fit with a single Boltzmann function. Figure 7: Measurement errors of dendritic HCN channels in cell-attached patches. ( a ) Intracellular voltage change ( V m ) evoked by ensemble HCN channel activity ( I C-A ) simultaneously recorded from the apical dendrite of a layer 5 pyramidal neuron (840 μm from the soma, separation between cell-attached and whole-cell pipette=10 μm). ( b ) Linear relationship between the amplitude of ensemble HCN channel activity in cell-attached patches and intracellular depolarization at apical dendritic sites of layer 5 pyramidal neurons. Data were gathered at room (23–24 °C, filled symbols) or near physiological (35–37 °C, open symbols) temperatures, and were fit by linear regression (lines). ( c ) Voltage-dependent activation of ensemble HCN channel activity ( I C-A ) in a cell-attached patch recorded from the apical dendrite of a layer 5 pyramidal neuron (850 μm from the soma). The lower traces show the intracellular voltage responses simultaneously recorded under whole-cell current-clamp ( V m ; 9 μm separation between pipettes). Note the generation of AP firing. ( d ) Pooled data demonstrating the linear relationship between HCN channel activity in cell-attached patches and intracellular depolarization, when measured at steady-state (filled symbols, fit by linear regression, line), but the minimal voltage deviation apparent at the peak of HCN tail currents (open symbols). Pooled data ( n =7) represent mean±s.e.m. ( e ) Transmembrane voltage corrected activation curve of apical dendritic HCN channels. Pooled data ( n =7, mean±s.e.m.) have been fit with a single Boltzmann function. Full size image Finally, to explore whether transient inward currents were distorted by transmembrane voltage changes, we recorded pharmacologically isolated sodium currents in cell-attached patches from the somata of TC neurons at room temperature. In contrast to the significant distortion of voltage-activated potassium and HCN channels, the amplitude and time course of ensemble sodium channel activity was found to be similar when recorded under whole-cell v-c and c-c recording conditions ( Fig. 8a,b ). We observed that the first sodium current of a train produced only a small intracellular voltage change ( Fig. 8c ) that temporally summated during the repetitive activation of ensemble sodium channel activity ( Fig. 8a ; V H =0 mV; pre-pulse=40 mV, 300 ms duration; pulse amplitude=−100 mV, duration=5 ms, inter-pulse interval=20 ms). These data indicate that the properties of transient ensemble sodium channel activity are faithfully reported by cell-attached recording techniques, consistent with the primary role of the fast sodium channels to rapidly charge the membrane capacitance, and not to produce long-lasting voltage deviations [48] . 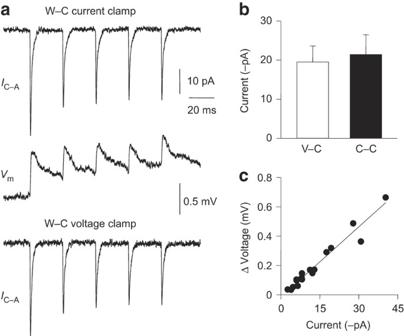Figure 8: Ensemble sodium channel activity is accurately reported in cell-attached patches. (a) Trains of ensemble sodium channel activity (IC-A) recorded in a cell-attached patch under simultaneous whole-cell current- and voltage-clamp conditions from the soma of thalamocortical neuron. The small intracellular voltage deviations recorded under whole-cell current-clamp (Vm) are shown. (b) Pooled data showing the similarity in the peak amplitude of ensemble sodium channel activity recorded in cell-attached patches under simultaneous voltage- (v-c) or current-clamp (c-c) conditions. Pooled data (n=7) represent mean±s.e.m. (c) Linear relationship between the peak amplitude of ensemble sodium channel activity in cell-attached patches and intracellular depolarization for the first current of each train. Data have been fit by linear regression (line). Figure 8: Ensemble sodium channel activity is accurately reported in cell-attached patches. ( a ) Trains of ensemble sodium channel activity ( I C-A ) recorded in a cell-attached patch under simultaneous whole-cell current- and voltage-clamp conditions from the soma of thalamocortical neuron. The small intracellular voltage deviations recorded under whole-cell current-clamp ( V m ) are shown. ( b ) Pooled data showing the similarity in the peak amplitude of ensemble sodium channel activity recorded in cell-attached patches under simultaneous voltage- (v-c) or current-clamp (c-c) conditions. Pooled data ( n =7) represent mean±s.e.m. ( c ) Linear relationship between the peak amplitude of ensemble sodium channel activity in cell-attached patches and intracellular depolarization for the first current of each train. Data have been fit by linear regression (line). Full size image Quantification of the properties and sub-cellular distribution of voltage-activated ion channels is a central problem in neuroscience, not least, because accurate and predictive computational models of single neurons and neuronal networks are reliant on this information. Cell-attached and cell-free patch-clamp techniques have become the methods of choice for the analysis of the functional properties and sub-cellular distribution of voltage-activated ion channels in central neurons [6] , [10] , [11] , [12] , [13] , [14] , [15] , [16] , [17] , [18] , [19] , [20] , [21] , [22] , [23] , [24] , [25] , [26] . Here, we report that the most non-invasive variant of the patch-clamp technique, cell-attached recordings [6] , suffer significant measurement errors of the properties (voltage dependence and kinetics) and the surface density of voltage-activated ion channels in central neurons. We find that these measurement errors arise because of the generation of transmembrane voltage changes produced by the flow of ionic current through voltage-activated ion channels in the tip of the cell-attached recording pipette. We demonstrate the magnitude of errors generated by transmembrane voltage changes by controlling the intracellular membrane potential using whole-cell v-c techniques. In this way, we directly observed the generation of a transmembrane current generated by ensemble voltage-activated ion channels in cell-attached patches, a finding supported by the report of mirror single receptor-operated channel currents simultaneously recorded at the cell-attached and whole-cell level in electrically compact neurons [49] . Measurement errors were pronounced for classes of voltage-activated channels that showed little inactivation, and were minimal for channels types, such as sodium channels, which exhibit rapid inactivation. The distortion of the kinetics and measurement of the surface density of voltage-activated ion channels in cell-attached patches, are of particular concern. We found, for example, that the time course and amplitude of ensemble potassium and HCN channel activity in cell-attached patches were significantly altered, with transmembrane voltage responses leading to the erroneous generation, or the exaggeration, of a transient component to ensemble potassium channel activity in TC and dopaminergic midbrain neurons. As potassium channel types, which underlie transient and sustained potassium currents are often apparent in cell-attached patches [1] , [10] , [11] , [27] , separation by simple kinetic analysis of cell-attached recordings cannot be relied on. The magnitude of measurement errors was dependent on the density of voltage-activated channels in cell-attached patches and the apparent input resistance of the neuron. Neurons or isolated cells with high apparent input resistance showed the greatest cell-attached measurement errors, as originally predicted by recording from isolated cells and membrane vesicles [31] , [32] , [33] , a finding that can be understood by Ohm's law. It should noted, however, that we observed significant errors in the measurement of ensemble channel activity in cell-attached patches recorded from central neurons maintained in acute brain-slices at room and near physiological temperatures ( Supplementary Fig. S3 ). Indeed, in large layer 5 pyramidal neurons, a neuronal class with a low apparent input resistance [46] , voltage errors significantly distorted the measurement of the density of voltage-activated channels at room and physiological temperatures. We suggest, by first approximation, that the magnitude of transmembrane voltage errors can be estimated by knowledge of the apparent input resistance of the neuron. Notably, modelling and experimental studies have suggested that apparent input resistance is not uniform throughout a neuron, because of morphological and electrotonic constraints [50] ; for example thin dendritic branches are predicted to have a high apparent input resistance. Our data suggest that cell-attached measurement errors will, in turn, be non-uniform; the apparent input resistance at the site of cell-attached recording should therefore be determined. Voltage deviations generated by ensemble channel activity were, however, not only shaped by the passive properties of neurons, but also influenced by the recruitment of other voltage-activated channels expressed by a neuron. This effect was most evident in neurons that generated action potential firing in response to ensemble channel activity in cell-attached patches. These findings highlight that in the unperturbed state, cell-attached recordings made with pipette contents designed to isolate the properties of a single ionic current can evoke whole-cell voltage changes that interact with the repertoire of ionic currents expressed by a neuron. In summary, we find that the generation of transmembrane voltage directly leads to errors in the measurement of the properties of ensemble voltage-activated ion channel activity in cell-attached recordings from central neurons. When taken together with measurement errors apparent for somatic whole-cell v-c recordings [9] , because of space-clamp limitations, these findings emphasize that knowledge of the potential measurement errors associated with common electrophysiological recording techniques are essential when choosing the appropriate technique to address a specific problem. Brain slice preparation Brain slices (300 μm) were prepared from Wistar rats (P20–P36) following Institutional and UK Home Office guidelines, and maintained in a solution containing (mM): 125 NaCl; 25 NaHCO 3 ; 3 KCl; 1.25 NaH 2 PO 4 ; 1 CaCl 2 ; 6 MgCl 2 , 3 Na pyruvate and 25 glucose. Brain slices were transferred to a recording chamber perfused with a solution of composition (mM): 125 NaCl; 25 NaHCO 3 ; 3 KCl; 1.25 NaH 2 PO 4 ; 2 CaCl 2 ; 1 MgCl 2 , 3 Na pyruvate and 25 glucose, bubbled with 95% O 2 /5% CO 2 , at room (23–25 °C) or near physiological (35–37 °C) temperature. In the majority of experiments, antagonists of excitatory and inhibitory amino-acid receptors were included in the extracellular media (6-cyano-7-nitroquinoxaline-2,3-dione (10 μM); 6-imino-3-(4-methoxyphenyl)-1(6H)-pyridazinebutanoic acid hydrobromide (10 μM); D -(−)-2-amino-5-phosphonopentanoic acid (50 μM)). Electrophysiological and imaging procedures Cell-attached v-c or simultaneous cell-attached and whole-cell recordings were made from the soma or dendrites of neurons visualized under infrared differential contrast microscopy. Somatic or dendritic cell-attached v-c recordings were made with an Axopatch 200B amplifier (Molecular Devices). Whole-cell recordings were made with an independent amplifier, either an Axopatch 200B or dedicated current-clamp amplifier (BVC-700A, Dagan), depending on the experimental design. For whole-cell v-c recordings series resistance was compensated by >80% in the presence of <10 μs lag. Whole-cell recording pipettes were filled with (mM): 135 K-gluconate; 10 HEPES; 7 NaCl; 2 Na 2 -ATP; 2 MgCl 2 ; 0.3 Na-GTP and 0.01 Alexa Fluor 568 (Molecular Probes) (pH 7.2–7.3, KOH). Cell-attached recording electrodes were filled with the same solution for experiments involving voltage ramps. For analysis of ensemble potassium channel activity, pipettes were filled with (mM): 125 NaCl; 10 HEPES; 3 KCl; 2 CaCl 2 ; 1 MgCl 2 ; 0.2 CdCl 2 and tetrodotoxin 0.001 (pH 7.3–7.4, NaOH). For cell-attached recording of pharmacologically isolated ensemble sodium channel activity, pipettes were filled with (mM): 125 NaCl; 30 tetraethylammonium chloride; 5 4-aminopyridine; 10 HEPES; 2 CaCl 2 ; 1 MgCl 2 ; 0.2 CdCl 2 (pH 7.2–7.3, NaOH), whereas for the recording of ensemble hyperpolarization-activated cyclic nucleotide (HCN)-gated channel activity, pipettes were filled with (mM): 120 KCl; 20 tetraethylammonium chloride; 10 HEPES; 5 4-aminopyridine; 3 BaCl 2 ; 2 CaCl 2 ; 1 MgCl 2 ; 1 NiCl 2 ; 0.5 CdCl 2 and 0.001 tetrodotoxin (pH 7.4, KOH). Voltage recordings were not corrected for liquid junction potentials. Whole-cell recording pipettes had a resistance of between 4 to 6 MΩ and pipettes for cell-attached recordings 8–10 MΩ. Current and voltage signals were low-pass filtered (DC to 10 KHz) and acquired at 30–50 KHz. For the cell-attached measurement of ensemble voltage-activated channel activity, other than that evoked by voltage-ramps, currents were subjected to offline leak subtraction, by the digital subtraction of leak currents generated in response to an interlaced and scaled (1/10) voltage command step. To ensure consistency, whole-cell recorded currents were subject to an identical leak subtraction procedure. Values of pipette command voltage are given in the text as delivered to the recording electrode, while cell-attached voltage command steps and recorded membrane currents have been inverted for illustration. Apparent input resistance was calculated form families of voltage deviations evoked by long (>200 ms) current steps under whole-cell c-c recording conditions. The maximum and minimum first and third quadrant steady-state current–voltage relationship were determined by linear regression. At the termination of each experiment, the location and morphology of neurons were examined by fluorescence microscopy and digitally recorded (Retiga EXI, Q Imaging). Data were acquired and analysed using AxographX software (AxographX). Numerical values in the text are presented as mean±s.e.m., and statistical analysis, analysis of variance and Student's t -test (two-tailed), was performed using Prism (GraphPad) software. Cell culture and transfection HEK293T cells, grown in poly- L -lysine-coated six-well plates, were transiently transfected with 0.4 μg mHCN1CFP/pECFP-Cl, which contained the full-length coding region of mHCN1 channel isoform conjugated at the amino terminus with a cyan florescent protein, using Effectene (Qiagen). Experiments were performed 48–72 h post-transfection. HEK293T cells were maintained in an extracellular solution (mM): 145 NaCl; 10 HEPES; 3 KCl; 2 CaCl 2 ; 1 MgCl and 10 glucose (pH 7.4, NaOH) in the recording chamber at room temperature. Simultaneous whole-cell and cell-attached recordings were made from isolated transiently transfected cells identified under fluorescence microscopy. How to cite this article: Williams, S.R. & Wozny, C. Errors in the measurement of voltage-activated ion channels in cell-attached patch-clamp recordings. Nat. Commun. 2:242 doi: 10.1038/ncomms1225 (2011).